Caloric restriction reduces age-related and all-cause mortality in rhesus monkeys Caloric restriction (CR) without malnutrition increases longevity and delays the onset of age-associated disorders in short-lived species, from unicellular organisms to laboratory mice and rats. The value of CR as a tool to understand human ageing relies on translatability of CR’s effects in primates. Here we show that CR significantly improves age-related and all-cause survival in monkeys on a long-term ~30% restricted diet since young adulthood. These data contrast with observations in the 2012 NIA intramural study report, where a difference in survival was not detected between control-fed and CR monkeys. A comparison of body weight of control animals from both studies with each other, and against data collected in a multi-centred relational database of primate ageing, suggests that the NIA control monkeys were effectively undergoing CR. Our data indicate that the benefits of CR on ageing are conserved in primates. The marked anatomical, physiological and behavioural similarities between humans and non-human primates make the latter uniquely suited for providing insights into the biology of human ageing. With advancing age, many of the familiar age-related phenotypes exhibited in humans are also observed in rhesus macaques ( Macaca mulatta ), including the redistribution of body fat, greying and thinning of hair, loss of vigour, loss of muscle tone and loss of skin tone [1] , [2] , [3] , [4] . In addition, there are increases in clinical manifestations of diseases and disorders including diabetes, neoplasia, sarcopenia, bone loss and immune function [4] , [5] , [6] , all conditions that increase in prevalence with advancing age in humans. Caloric restriction (CR) is one of the most robust interventions shown to delay ageing in diverse species from yeast to mammals. Reduced calorie intake without malnutrition extends lifespan in rodents and delays the onset of multiple age-associated diseases [7] . Until recently, it was an open question whether the beneficial effects of CR are conserved in primates. Over the past twenty plus years, substantial data have been generated that support the concept that CR improves health in rhesus monkeys [8] , [9] . The first report on survival arose from the University of Maryland study where a 2.6-fold increased risk of death in control animals compared with restricted animals was reported in a study [10] ; however, the analysis was based on 109 ad libitum -fed animals including insulin-resistant and diabetic animals and only 8 animals on CR. In the University of Wisconsin (UW) adult-onset rhesus monkey CR study involving 76 animals, CR delayed disease onset and mortality in rhesus monkeys with 2.9-fold increased risk of disease and 3.0-fold increased risk death for control animals compared with CR animals [11] . In a parallel study of 120 animals conducted at the National Institute on Ageing (NIA), improvements in the health of CR animals did not reach significance ( P =0.06) and survival was not significantly different between control-fed and CR monkeys in their cohorts [12] . The contrasting results from these studies raise an important issue for biology of ageing research. In the past decade, studies conducted in shorter-lived species have provided valuable insights into the actions of CR and the mechanisms by which it impinges on ageing. We now know that CR induces an active response rather than a passive mechanism of slower ageing, and a number of strong candidates have emerged as playing a central role in CR’s actions [13] , [14] , [15] . The translatability of these findings to human ageing is compromised if CR’s effect on ageing is not conserved. Here we show that adult-onset CR has positive impact on both age-related and overall survival in rhesus monkeys and show that the beneficial impact of CR on non-human primate ageing is a point of agreement between the UW and NIA studies. Rhesus monkey ageing and CR study For rhesus monkeys in captivity, median survival is ~26 years of age, 10% survival is ~35 years of age and maximum survival is ~40 years of age [8] . The rhesus monkey CR and ageing study was initiated in 1989 at the Wisconsin National Primate Research Center (WNPRC) [16] . Animals were recruited in two phases, the first containing 30 males and the second phase, begun in 1994, in which 30 females and an additional 16 males were added. Animals in all groups were adults when introduced into the study (7–14 years old). The classic rodent CR experiment, in which lifespan may be extended by as much as 40% [17] , involves animals being placed on the diet at an early age just after weaning. Despite initial uncertainties as to whether adult-onset CR would also prove beneficial in terms of lifespan, careful studies have shown that with gradual reduction in food intake adult-onset of CR is almost as effective as early-onset in extending lifespan in rodents [18] . The adult-onset CR model was chosen for the rhesus monkey study on the basis that any potential ageing intervention in human studies would be initiated in adult populations. Within each of the three groups, animals were randomized to control or CR diets taking into consideration baseline food intake, body weight and age. Individualized food allotments were calculated based on daily food intake data that were collected for each animal over a 3–6-month period before initiation of the dietary intervention. For each animal in the CR groups, the individual intake determined at baseline was reduced by 10% per month over a 3-month period to reach the desired 30% restriction. CR reduces age-related and all-cause mortality To assess the impact of CR on age-related and all-cause survival, the cause of death for each monkey was determined on necropsy by a board-certified pathologist who was blinded to the animal’s diet group. Deaths due to acute conditions clinically unrelated to ageing were excluded from the age-related mortality analysis but were retained for the evaluation of all-cause mortality. Of the original 76 animals, 63% (24/38) of the control animals died of age-related causes compared with only 26% (10/38) of the CR group. Considering only age-related deaths and excluding animals with non-age-related deaths (NARDs), a statistically significant effect of CR in increasing survival was observed (Cox regression P =0.007; Fig. 1a ) with a hazard ratio (HR) of 2.89 (95% confidence interval (CI): 1.34–6.25) indicating that at any point in time the control animals had 2.9 times the rate of death from an age-related cause when compared with animals under CR. Conducting this same analysis including NARDs but treating them as censored values also revealed a statistically significant effect of CR in increasing survival (Cox regression P =0.001) with a HR of 3.63 (95% CI: 1.69–7.81). 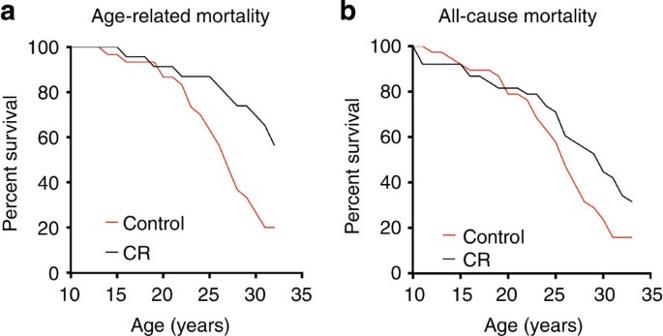Figure 1: Mortality curves. (a) Age-related mortality. Animals that died from non-age-related causes are excluded. The Cox regression detected a statistically significant effect of CR in increasing survival (P=0.007) with a HR of 2.89 (95% CI: 1.34–6.25). (b) All-cause mortality. These curves depict data for all animals on the study not censored for cause of death. The Cox regression detected a statistically significant effect of CR (P=0.037;Fig. 1b) with an estimated HR of 1.78 (95% CI: 1.04–3.04). Figure 1: Mortality curves. ( a ) Age-related mortality. Animals that died from non-age-related causes are excluded. The Cox regression detected a statistically significant effect of CR in increasing survival ( P =0.007) with a HR of 2.89 (95% CI: 1.34–6.25). ( b ) All-cause mortality. These curves depict data for all animals on the study not censored for cause of death. The Cox regression detected a statistically significant effect of CR ( P =0.037; Fig. 1b ) with an estimated HR of 1.78 (95% CI: 1.04–3.04). Full size image Survival analysis showed that effect of CR on all-cause mortality is also statistically significant (Cox regression P =0.037; Fig. 1b ) with an estimated HR of 1.78 (95% CI: 1.04–3.04) indicating that at any point in time the control animals had 1.8 times the rate of death from any cause when compared with animals under CR. In all, 8 controls and 16 animals subjected to CR died of non-age-related causes, which included complications of anaesthesia, gastric bloat, endometriosis and injury. Although twice as many CR animals died from a NARD, there were twice as many CR animals alive at this stage of the study. For animals younger than 20 years of age the incidence of NARD was 11% for control animals and 13% for CR. A competing risk model that treated age-related and non-age-related deaths as mutually exclusive events indicated that CR animals were not significantly more likely to die from a non-age-related cause (competing risk model P =0.373). Applying the same analysis to age-related deaths confirmed the previous result of the censored analysis, in that the effect of CR on age-related mortality was statistically significant (competing risk model P =0.001) with HR of 3.62 (95% CI: 1.69–7.82). Differences in survival of the CR and control animals are shown in Table 1 . Estimates of lifespan were determined using the Kaplan–Meier statistical model and parametric survival analysis assuming a Weibull distribution, with both indicating improved survival for monkeys on CR. Importantly, the median survival of control animals (~26 years) is comparable to that of animals at WNPRC not participating in this study, demonstrating that CR has increased survival relative to normal rhesus monkey ageing. Table 1 Estimates of lifespan. Full size table Comparison of control monkeys from UW and NIA CR studies Recently, the results of the NIA rhesus monkey young-onset and old-age-onset CR study were published [12] , and although modest benefits in overall measures of health and function were observed in CR animals compared with controls, a significant difference in survival was not detected. To try to understand the differences in outcome, we focused on the differences in the study design. The implementation of the CR diet is a major point of divergence between the UW and NIA studies. The primary goals of the UW study were to investigate rhesus monkeys as a model for human ageing and to determine the impact of CR on ageing. The UW control animals were ad libitum fed to mirror human feeding habits. The NIA study is closer to the classic CR study design used in rodent studies; the study included early-onset cohorts and NIA control animals were fed according to regulated portioning rather than ad libitum . We compared body weight data for control animals from the NIA study that had been previously published [19] , [20] with age- and gender-matched control animal data from the UW study ( Fig. 2a ). NIA female monkeys weighed significantly less than UW controls both at 12–18 and 21–25 years of age (Welch’s t -test P =0.014, P =0.049). Male monkeys of 10–12 years age from the NIA study also weighed less than those from the UW study (Welch’s t -test P =0.003). The body weight difference between an older age group of males showed the same trend but was not statistically significant (24–33 years, Welch’s t -test P =0.169); however, the reduced size of both cohorts ( n =7 NIA and n =4 UW) and the large variance among individuals at advanced age limits the possibility that statistical significance could be observed. 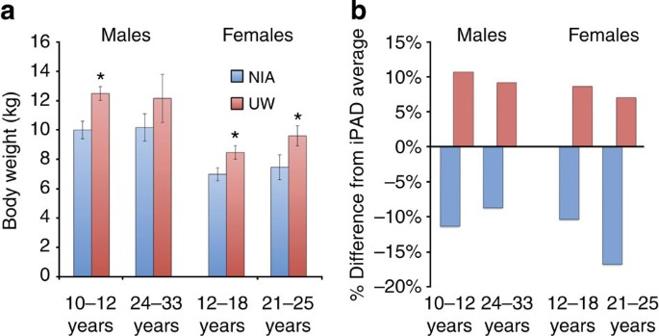Figure 2: Body weight comparisons. (a) Body weights for male and female control animals from UW and NIA studies. Males, 10–12 years: NIA=6, UW=15; 24–33 years: NIA=7, UW=4. Females, 12–18 years: NIA=20, UW=15; 21–25 years: NIA=5, UW=8. Data are shown as average±s.e.m. *P<0.05 (Welch’st-test). (b) Comparison of body weights for control animals on UW and NIA rhesus monkey ageing and CR studies with national averages for age- and gender-matched animals. Data shown in (a) are presented as per cent deviation from averages for males aged 10–12 years (175 animals, 2,790 data points), males aged 24–33 years (114 animals, 11,805 data points), females aged 12–18 years (334 individuals, 18,626 data points) and females aged 21–25 years (255 animals, 15,666 data points). Figure 2: Body weight comparisons. ( a ) Body weights for male and female control animals from UW and NIA studies. Males, 10–12 years: NIA=6, UW=15; 24–33 years: NIA=7, UW=4. Females, 12–18 years: NIA=20, UW=15; 21–25 years: NIA=5, UW=8. Data are shown as average±s.e.m. * P <0.05 (Welch’s t -test). ( b ) Comparison of body weights for control animals on UW and NIA rhesus monkey ageing and CR studies with national averages for age- and gender-matched animals. Data shown in ( a ) are presented as per cent deviation from averages for males aged 10–12 years (175 animals, 2,790 data points), males aged 24–33 years (114 animals, 11,805 data points), females aged 12–18 years (334 individuals, 18,626 data points) and females aged 21–25 years (255 animals, 15,666 data points). Full size image Comparison of CR studies with national monkey ageing data To place these data in a broader context, we next determined how the control animals from both studies compared with the national average for body weight for male and female rhesus monkeys within these age groups. The internet Primate Ageing Database (iPAD; http://ipad.primate.wisc.edu/ ) is a joint initiative of the NIA (intramural and extramural programs), NIH Office of Research Infrastructure Programs (ORIP) and the National Primate Research Center at the University of Wisconsin–Madison. The iPAD hosts clinical and biometric data from healthy, non-experimental, captive non-human primates housed in research facilities across the USA. Body weight averages of age- and gender-matched animals were calculated on the basis of iPAD data from 878 individuals using 48,887 data points ( Fig. 2b ). Although UW and NIA intramural studies both exclusively housed animals individually, the iPAD does not distinguish between group and individual housing so that data from iPAD included in comparison with UW and NIA intramural studies were not limited to individually housed animals. For each gender and age group, the UW control animals consistently weighed more than average. In contrast, the body weights of the NIA control animals were consistently lower than average for both genders and at both age groups considered. One explanation for the lack of difference in survival among animals from the NIA study is that the control animals were in fact restricted and the advantages of mild restriction on survival in the control animals were not improved by further restriction in the CR group. Data from the NIA old-age-onset male cohort is consistent with improved survival in both control and CR groups. Of the 20 male monkeys initiated into the study in old age, 5 lived beyond 40 years of age, 1 from the control group and 4 from the CR group. In over three decades of maintaining an ageing colony of >100 animals at the WNPRC, only one monkey with a known birth date reached 40 years of age. Furthermore, of the 3264 rhesus monkeys (175,456 data points) in the iPAD only two 40-year-old animals have been documented. These data indicate that the five 40-year-old monkeys from the NIA intramural study are exceptionally long-lived. CR studies encompass two central issues of relevance to human health, first the relationship between chronological age and increased disease incidence, and second how nutritional inputs can modulate ageing. To fully assess the impact of CR on non-human primate ageing both age-related and all-cause mortality must be considered. At the outset of the study it was not a foregone conclusion that CR would be beneficial in long-lived species, furthermore, there was some concern that CR may even be detrimental. Negative effects of CR have been reported in genetically diverse strains of mice [21] , and it has become apparent that there are strain-specific considerations in avoiding malnutrition while reducing calories. Our data show that while both age-related and all-cause survival are significantly improved with CR, there was no effect of CR on NARD. Although twice as many CR animals died of NARD compared with controls, the relative incidence of NARD between control and CR animals was not different and the risk of NARD was not different. These data argue against a negative impact of CR as implemented in this study. Estimates of median survival also reveal differences between control and CR animals. Medians for all-cause deaths are lower than that for age-related deaths but in both cases the estimated median lifespan of control animals was less than that of CR. As would be predicted from a delayed ageing model, a significant impact of CR on all-cause survival was apparent only at advanced ages. Compared with controls there are currently twice as many CR monkeys still alive (6 and 12, respectively), suggesting that the effect of CR in improving survival is likely to be sustained as the study draws to a close. The difference in outcomes of the UW and NIA monkey CR studies has raised questions about the relevance of insights gleaned from CR for human ageing and human health. The duration and costs of conducting a long-term CR study in monkeys make it likely that these experiments will not be repeated so it is essential to understand how two studies with similar objectives could report disparate findings with regard to survival and health. Using published data from the NIA study, we identified equivalent time points in data from the UW study and found significant differences in body weight between controls from the two studies. This suggests that compared with UW animals the NIA controls were modestly restricted. Furthermore, in comparison with a large data set from iPAD we find that NIA monkeys weigh less than the average monkey in captivity for both genders and at both ages investigated. The lack of difference between NIA controls and CR suggests that for primates there may be little advantage of moderate CR over modest CR—this would be an extremely important discovery and one that merits further investigation. A comprehensive analysis of non-human primate CR data generated at both UW and NIA sites is warranted. In addition to the differences in age of onset and feeding protocols, other important points of difference between the studies include diet composition (UW diet was purified and high in sucrose content) and genetic origin of the monkeys (Indian at UW, Chinese and Indian at NIA). It is highly likely that factors important in ageing that are not evident in either study independently will emerge from the analysis of the aggregate data. A major advantage of the non-human primate CR studies is the ability to determine primate-specific aspects of ageing and the role of nutrition in ageing. Biometrics, food intake, the environment and clinical histories of the animals are documented in detail. Similar data are available for human studies but the opportunity to investigate tissue-specific and cellular responses to age and diet is unparalleled. The monkey studies are the lynchpin connecting mechanistic studies in rodents and invertebrates to the more clinically constrained human studies. Given the conserved effect of CR on health and survival, we contend that the rhesus monkey CR and ageing model is an important resource to test the conservation of roles of putative longevity factors identified in studies of short-lived animals and the likelihood that these advances will translate directly to human ageing and human health. Animals and diets The ageing and CR study was initiated in 1989 at the WNPRC. All animals were of Indian origin, were born at the WNPRC and were adults (7–14 years old) when introduced into the study. Complete clinical and experimental histories are maintained for each animal. Before the start of this experiment, no animal had any clinical or experimental history that would be expected to affect disease susceptibility or mortality. Initially, the study included 30 males and the cohort was expanded in 1994 to include an additional 30 females and 16 males. The animals were evenly matched and randomized to control or CR diets taking into consideration baseline food intake, body weight and age. Individualized food allotments were calculated on the basis of daily food intake data that had been collected for each animal over a 3–6-month period before the start of this study. Once animals were assigned to either control or CR group, each CR animal’s individually determined baseline intake was reduced by 10% per month over a 3-month period to reach the desired 30% restriction. Animals were fed a semi-purified, nutritionally fortified, low-fat diet containing 15% protein and 10% fat. As part of the study design, animals were treated for presenting conditions. For example, diabetics receive insulin sensitizers or insulin, animals with diverticulosis receive fibre supplements and females with endometriosis were treated with hormone suppression. This study was conducted in accordance with protocols approved by the University of Wisconsin–Madison Graduate School Institutional Animal Care and Use Committee. Survival analysis The mortality analysis performed included all animals with known diagnoses or cause of death before 10 October 2013. To determine the effect of CR on mortality, a Cox proportional hazards (PH) regression with sex and group (CR or control) as predictors was used to estimate the survival and hazard functions. For those whose deaths were not age associated, animals were censored and their age at death was used as the time variable in the Cox regressions. The PH assumption was tested by fitting a non-PH Cox regression with a CR by time interaction. For both age-related and all-cause mortality analysis the interaction was not significant, and thus, PH models were considered valid. We also performed a competing risks model that treated age-related and non-age-related deaths as mutually exclusive events compared with neither event occurring (that is, animals still alive and censored). These events are considered competing risks in that if an animal dies from a non-age-related cause they are no longer at-risk for an age-related death (and vice versa). We also estimated median and mean lifespan using Kaplan–Meier and parametric survival analysis assuming a Weibull distribution. Body weight comparison Data were obtained from NIA published reports and corresponding data from age- and gender-matched animals from the UW study were acquired from unpublished health records. Comparisons between the NIA and UW study were performed using Student’s t -test. National averages for body weights were calculated using data from the iPAD. Comparisons of body weight from the NIA and UW studies to iPAD data were performed with Welch’s t -test in light of inequalities in sample size and variance. How to cite this article: Colman, R. J. et al. Caloric restriction reduces age-related and all-cause mortality in rhesus monkeys. Nat. Commun. 5:3557 doi: 10.1038/ncomms4557 (2014).